Efficient purification of ethene by an ethane-trapping metal-organic framework Separating ethene (C 2 H 4 ) from ethane (C 2 H 6 ) is of paramount importance and difficulty. Here we show that C 2 H 4 can be efficiently purified by trapping the inert C 2 H 6 in a judiciously designed metal-organic framework. Under ambient conditions, passing a typical cracked gas mixture (15:1 C 2 H 4 /C 2 H 6 ) through 1 litre of this C 2 H 6 selective adsorbent directly produces 56 litres of C 2 H 4 with 99.95%+ purity (required by the C 2 H 4 polymerization reactor) at the outlet, with a single breakthrough operation, while other C 2 H 6 selective materials can only produce ca . ⩽ litre, and conventional C 2 H 4 selective adsorbents require at least four adsorption–desorption cycles to achieve the same C 2 H 4 purity. Single-crystal X-ray diffraction and computational simulation studies showed that the exceptional C 2 H 6 selectivity arises from the proper positioning of multiple electronegative and electropositive functional groups on the ultramicroporous pore surface, which form multiple C–H···N hydrogen bonds with C 2 H 6 instead of the more polar competitor C 2 H 4 . As the most important chemical product, ethene (C 2 H 4 ) is generally obtained through steam cracking and thermal decomposition of naphtha or ethane (C 2 H 6 ) (ref. 1 ). Besides being obtained as a byproduct of petroleum refining, C 2 H 6 is also isolated on an industrial scale from natural gas (CH 4 70 ∼ 96%, C 2 H 6 1 ∼ 14% and CO 2 0 ∼ 8%) (ref. 2 ). As a result of their similar physical properties, it is difficult to separate C 2 H 6 , C 2 H 4 and CO 2 (refs 3 , 4 , 5 ). In industry, C 2 H 6 and C 2 H 4 are separated by cryogenic high-pressure distillation, typically at 7–28 bar and 183–258 K using very high towers consisting of over 150 trays, which is very energy consuming (7 GJ t −1 ) and constitutes a notable portion of the ethylene cost [6] , [7] . To save energy, separation methods effective at the ambient temperature and pressure are highly demanded [8] , [9] , [10] , [11] . Passing the gas mixture through a fixed-bed adsorber can be a very simple and promising approach to afford low energy consumption and high product purity. Because unsaturated hydrocarbons like to coordinate with metal ions, C 2 H 4 can be selectively bound and separated from its saturated counterpart C 2 H 6 (refs 12 , 13 , 14 , 15 , 16 ). Compared with other types of porous materials, porous metal-organic frameworks (MOFs) are unique for their diversified/designable framework structures and pore surfaces, including the ease of introducing open metal sites (OMSs), which have shown great potentials for C 2 H 4 /C 2 H 6 separation [17] , [18] , [19] , [20] , [21] , [22] . In the fix-bed separation process, the un-adsorbed C 2 H 6 first breakthrough, and C 2 H 4 enriched in the stationary phase is later obtained by heating and/or inert-gas blowing. Because the un-adsorbed C 2 H 6 residing in the mobile phase contaminates the desired product C 2 H 4 during the desorption stage, the highest C 2 H 4 purity produced by a full adsorption–desorption cycle can just reach 99%+ (refs 13 , 17 , 23 , 24 ), and at least four such cycles are necessary to achieve 99.95%+ (ref. 25 ), the lower limit required by the C 2 H 4 polymerization reactor [26] , [27] , [28] . Obviously, this problem can be solved by using a C 2 H 6 selective adsorbent, which not only improves the C 2 H 4 purity but also reduces energy consumption. The simple separation operation and device (just one adsorption process in a single breakthrough operation) are also necessary for onsite supply of purified C 2 H 4 . However, such an unusual adsorption behaviour has been only reported for a few low-polarity or hydrophobic MOFs [29] , [30] , [31] , [32] , [33] , [34] , [35] , [36] , and their C 2 H 4 /C 2 H 6 separation performances (that is, C 2 H 6 /C 2 H 4 selectivities) are poor, because the polarities of C 2 H 4 and C 2 H 6 are very similar and can be hardly distinguished by hydrophobic adsorbents. 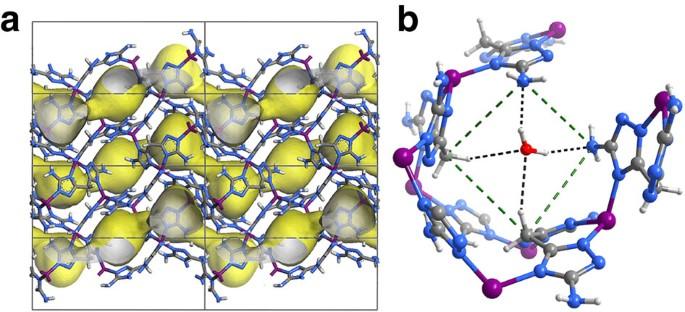Figure 1: X-ray crystal structure of MAF-49·H2O. (a) Framework (Zn purple, C dark grey, H light grey, N blue) and pore surface (yellow/grey curved surface) structures. Guest molecules are omitted for clarity. (b) Local environment and hydrogen-bonding interactions of the narrowest channel neck (highlighted by green dashed lines). As C 2 H 6 possesses the lowest polarity (quadrupole moment) compared with similar molecules such as C 2 H 4 and CO 2 ( Supplementary Table 1 ) [37] ; polar adsorbents are generally selective for the latter gases. However, considering that the electropositive and electronegative portions locate quite differently among these gas molecules, we speculated that by rational utilization of polar functional groups, it is still possible to design a MOF with optimized pore size/shape and surface electrostatic distribution that can bind C 2 H 6 much stronger than for C 2 H 4 . Herein, we report the design, structure and gas adsorption/separation properties of such a C 2 H 6 -trapping MOF, which is useful for not only direct producing highly pure C 2 H 4 from C 2 H 4 /C 2 H 6 mixtures, but also efficient separation of four-component CH 4 /C 2 H 4 /C 2 H 6 /CO 2 mixtures and extraction of C 2 H 6 from natural gas. Synthesis, structure and stability Bis(5-amino-1 H -1,2,4-triazol-3-yl)methane (H 2 batz) with two 3-amino-1,2,4-triazole rings bridged by a methylene group was designed as a new ligand combining multiple nitrogen atoms as hydrogen-bonding acceptors and methylene groups as dipole repulsion groups, as well as short bridging lengths for construction of an ultramicroporous framework. Reaction of H 2 batz and Zn(OH) 2 in dilute aqueous ammonia produced a porous metal-azolate framework [Zn(batz)]·0.5H 2 O (MAF-49·H 2 O). 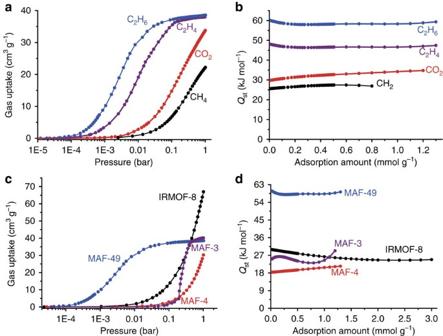Figure 2: Single-component gas adsorption properties. (a) Gas adsorption isotherms for C2H6, C2H4, CO2and CH4in MAF-49 at 316 K. (b) The coverage-dependent C2H6, C2H4, CO2and CH4adsorption enthalpy obtained by the Virial method. (c) C2H6adsorption isotherms of MAF-49, MAF-3, MAF-4 and IRMOF-8 measured at 316 K. (d) Coverage-dependent C2H6adsorption enthalpy of MAF-49, MAF-3, MAF-4 and IRMOF-8. Single-crystal X-ray diffraction (SCXRD) analysis of MAF-49·H 2 O ( Supplementary Table 2 and Supplementary Data 1 ) showed that each Zn(II) is tetrahedrally coordinated by four triazolate nitrogen atoms from three batz 2– ligands ( Supplementary Fig. 1 ), and each batz 2– ligand coordinates to three Zn(II) ions in a bisimidazolate mode, giving a three-dimensional (3D) coordination framework with narrow 1D zigzag channels ( Fig. 1a ). Since only four of the eight nitrogen donors of batz 2– are utilized according to the coordination requirement of Zn(II), the pore surface of MAF-49 is rich with electronegative nitrogen atoms, although some of them form intra-framework N–H···N hydrogen bonds to reduce their abilities as hydrogen-bonding acceptors. Notably, the narrowest section of the 1D channel (3.3 × 3.0 Å 2 ) is approximately a folded four-membered ring defined by a pair of free amino groups (with their lone electron pairs) and a pair of methylene groups with a cis -configuration, which is occupied by a guest H 2 O molecule with two O–H···N and two C–H···O hydrogen bonds ( Fig. 1b ). Figure 1: X-ray crystal structure of MAF-49·H 2 O. ( a ) Framework (Zn purple, C dark grey, H light grey, N blue) and pore surface (yellow/grey curved surface) structures. Guest molecules are omitted for clarity. ( b ) Local environment and hydrogen-bonding interactions of the narrowest channel neck (highlighted by green dashed lines). Full size image Thermogravimetry and powder XRD showed that MAF-49·H 2 O can be readily activated and is stable to 450 °C in nitrogen ( Supplementary Fig. 2 ), in boiling water for at least 1 month and in aqueous acid/base (4≤pH≤12) at room temperature for at least 1 week ( Supplementary Fig. 3 ), which is extraordinary among MOFs and can be partly explained by the strong metal-azolate coordination bonds [38] . SCXRD showed that complete dehydration leads to a slight framework expansion (0.17% in volume, Supplementary Table 2 and Supplementary Data 2 ). Gas adsorption property and mechanism Single-component adsorption isotherms for CH 4 , C 2 H 6 , C 2 H 4 and CO 2 were measured for guest-free MAF-49 at 298 K, 307 K and 316 K ( Fig. 2a and Supplementary Fig. 4 ). According to their different isotherm shapes, it can be judged that the host–guest binding follows C 2 H 6 >C 2 H 4 >CO 2 >CH 4 . The gas adsorption enthalpies were calculated quantitatively by Virial analyses ( Fig. 2b and Supplementary Fig. 5 ), which are 60 kJ mol −1 , 48 kJ mol −1 , 30 kJ mol −1 and 25 kJ mol −1 for C 2 H 6 , C 2 H 4 , CO 2 , and CH 4 , respectively, at zero-coverage. The mixed gas adsorption isotherms for equimolar C 2 H 6 /C 2 H 4 , C 2 H 6 /CO 2 and C 2 H 6 /CH 4 mixtures were simulated by the ideal adsorbed solution theory [39] , in which the single-component adsorption isotherms were fitted by the Langmuir−Freundlich model ( Supplementary Fig. 6 ). At total pressure of 100 kPa and a temperature of 316 K, the C 2 H 6 /C 2 H 4 , C 2 H 6 /CO 2 and C 2 H 6 /CH 4 selectivities of these mixtures were calculated as ca . 9, 40 and 170, respectively ( Supplementary Fig. 7 ). Notably, the C 2 H 6 /C 2 H 4 selectivity of MAF-49 is much higher than the highest value in the literature (2.4 for IRMOF-8 at 318 K) (ref. 31 ). Except for CH 4 with obviously lower molecular weight and boiling point, which interacts weakly with all adsorbents, the binding strength order of MAF-49 for other three heavier gases is unusual. Among a variety of physical properties of the four gases, only the polarizability trend is consistent with the binding trend ( Supplementary Table 1 ). Nevertheless, the small differences of their polarizabilities are not enough to explain the large variation of their adsorption enthalpies, especially for C 2 H 6 and C 2 H 4 . Notably, the C 2 H 6 adsorption enthalpy is significantly higher than reported values, while the C 2 H 4 one is moderate [18] . Figure 2: Single-component gas adsorption properties. ( a ) Gas adsorption isotherms for C 2 H 6 , C 2 H 4 , CO 2 and CH 4 in MAF-49 at 316 K. ( b ) The coverage-dependent C 2 H 6 , C 2 H 4 , CO 2 and CH 4 adsorption enthalpy obtained by the Virial method. ( c ) C 2 H 6 adsorption isotherms of MAF-49, MAF-3, MAF-4 and IRMOF-8 measured at 316 K. ( d ) Coverage-dependent C 2 H 6 adsorption enthalpy of MAF-49, MAF-3, MAF-4 and IRMOF-8. Full size image To elucidate the very different C 2 H 6 , C 2 H 4 and CO 2 affinities of MAF-49, their preferential host–guest structures and energy changes were calculated by grand canonical Monte Carlo simulation and further periodic density functional theory optimization. The obtained binding energies of the final host–guest structures are −56.7, −45.5 and −41.3 kJ mol –1 for C 2 H 6 , C 2 H 4 and CO 2 , respectively. However, to adsorb these gas molecules, the host framework undergoes different structural distortions from the guest-free form and consumes energies of +0.2 kJ mol –1 , +0.3 kJ mol –1 and +5.6 kJ mol –1 , respectively. 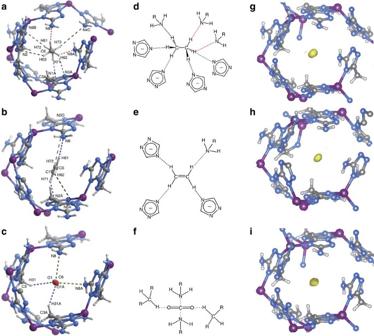Figure 3: Host–guest fittings and interactions. Preferential adsorption sites for (a) C2H6, (b) C2H4and (c) CO2in MAF-49 revealed by computational simulations (Zn purple, C dark grey, H light grey, N blue). Schematic representation of the corresponding host–guest interactions for (d) C2H6, (e) C2H4and (f) CO2. Strong (H···N/O<2.3 Å), weak (2.3 Å<H···N/O<2.8 Å) and almost negligible (H···N/O>2.8 Å) C–H···N interactions are displayed as red, blue and black dashed lines, respectively. 3D electron density maps (Fo–Fccontoured at 0.80 e Å−3in yellow) of MAF-49 loaded with trace amounts of (g) C2H6, (h) C2H4and (i) CO2. Taking both the host–guest binding and host-framework distortion into consideration, the total energies or adsorption enthalpies can be calculated as −56.5 kJ mol –1 , −45.2 kJ mol –1 and −35.7 kJ mol –1 for C 2 H 6 , C 2 H 4 , and CO 2 , respectively, which are consistent with the experimental values ( Supplementary Table 3 ). In the density functional theory optimized host–guest structures, it can be seen that C 2 H 6 , C 2 H 4 and CO 2 are all adsorbed in or very close to the narrowest channel neck, but they interact very differently with the pore surface. C 2 H 6 forms three strong C–H···N hydrogen bonds and three weak C–H···N electrostatic interactions with MAF-49 ( Fig. 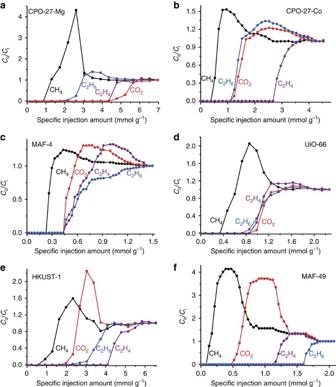Figure 4: Four-component gas mixture separation. Breakthrough curves of CH4/CO2/C2H4/C2H6mixture (1:1:1:1 (vol)) for (a) CPO-27-Mg, (b) CPO-27-Co, (c) MAF-4, (d) UiO-66, (e) HKUST-1 and (f) MAF-49 measured at 313 K and 1 bar. Lines are drawn to guide eyes.CiandCoare the concentrations of each gas at the inlet and outlet, respectively. 3a,d , Supplementary Table 4 ). Specifically, one methyl group interacts with two amino groups and an coordinated triazolate nitrogen atom of the narrowest channel neck, forming one very short and directional (C6-H61···N8) and one unsymmetrical-bifurcated/three-centred (C6-H62···N8A/N3A) hydrogen bonds, in which the H···N separations (2.15 Å) are much shorter than the sum of van der Waals radii of nitrogen (1.55 Å) and hydrogen (1.20 Å) atoms. The third strong hydrogen bond involves the hydrogen atom (H71) of another methyl group and a coordinated triazolate nitrogen atom (C8-H71···N1A), which is approximately centro-symmetric with the strongest one (C6-H61···N8) about the molecular centre and fits well with the most stable stagger conformation of C 2 H 6 . Besides, the less polar part of the pore surface, that is, two methylene groups of the batz 2– ligand (C3), fits well with the guest C 2 H 6 molecule in the context of both molecular shape and electrostatic potential. Figure 3: Host–guest fittings and interactions. Preferential adsorption sites for ( a ) C 2 H 6 , ( b ) C 2 H 4 and ( c ) CO 2 in MAF-49 revealed by computational simulations (Zn purple, C dark grey, H light grey, N blue). Schematic representation of the corresponding host–guest interactions for ( d ) C 2 H 6 , ( e ) C 2 H 4 and ( f ) CO 2 . Strong (H···N/O<2.3 Å), weak (2.3 Å<H···N/O<2.8 Å) and almost negligible (H···N/O>2.8 Å) C–H···N interactions are displayed as red, blue and black dashed lines, respectively. 3D electron density maps ( F o – F c contoured at 0.80 e Å −3 in yellow) of MAF-49 loaded with trace amounts of ( g ) C 2 H 6 , ( h ) C 2 H 4 and ( i ) CO 2 . Full size image For C 2 H 4 , two less strong C–H···N hydrogen bonds and two very weak C–H···N electrostatic interactions were observed ( Fig. 3b,e and Supplementary Table 4 ). The strongest one involves one methylene group and one amino group at the narrowest channel neck (C6-H61···N8), while the secondary one involves another methylene group and an uncoordinated triazolate nitrogen atom (C7-H71···N2A), which are also approximately centro-symmetric about the molecular centre. These two C–H···N hydrogen bonds are similar in geometry with the first and third strongest ones for C 2 H 6 . However, their H···N separations (2.54–2.65 Å) are obviously longer, albeit C 2 H 4 is more polar ( Supplementary Table 4 ). The cis -configuration of the two electronegative amino groups and two electropositive methylene groups of the narrow channel neck is crucial for the very different host–guest interactions. Obviously, the molecular geometry of C 2 H 4 prevents the two hydrogen atoms of a methylene group to form two strong hydrogen bonds with the narrow channel neck like H 2 O and C 2 H 6 . Furthermore, there is significant steric hindrance and electrostatic repulsion between the two C–H moieties of the two methylene groups from the host channel neck and the guest C 2 H 4 (C3···C6=3.88 Å, Supplementary Fig. 8 ), which pushes the guest away from the best position for forming a strong C–H···N hydrogen bond with the p -position amino group. Conversely, the methylene group of the host channel neck fits well with the threefold symmetric methyl group of C 2 H 6 ( Fig. 3a ). For the less strong C–H···N hydrogen bonds and other weak electrostatic attractive interactions, C 2 H 6 also fits much better with the locations of the electronegative nitrogen atoms, as compared with those for C 2 H 4 ( Fig. 3 and Supplementary Table 4 ). These observations indicate that the proper locations of both the electronegative nitrogen atoms and the electropositive methylene groups play critical roles in distinguishing C 2 H 6 and C 2 H 4 with large adsorption enthalpy difference. In the simulated host–guest structure for CO 2 , the guest carbon atom locates exactly at the centre of host channel neck, forming short contacts with two free amino groups simultaneously (N···C=2.91 Å), while two oxygen atoms of CO 2 interact with two methylene groups, respectively, through weak C–H···O hydrogen bonds (C···O=3.33, H···N=2.45 Å, ∠ C–H···N=135°) ( Fig. 3c,f , Supplementary Table 4 ). Although these host–guest interactions seem relatively strong, the channel neck diameter (measured by the separation of the p -position amino and methylene groups, N8···C3 3.60 Å) significantly expanded from the guest-free state (3.13 Å), while it changes little after loading C 2 H 6 (3.18 Å) and C 2 H 4 (3.31 Å), indicating that there is significant steric hindrance and repulsive effect between the CO 2 molecule and the host framework, and the very short C···N separation is actually the result enforced by the contraction action of the channel neck ( Supplementary Fig. 9 ). It should be noted that all carbon atoms of C 2 H 6 and C 2 H 4 reside on one side of the quadrangular channel neck, resulting in much smaller steric hindrance effects compared with CO 2 ( Supplementary Fig. 10 ). To confirm the simulation results and directly visualize the host–guest interactions, we carried out SCXRD analyses for MAF-49 loaded with trace amounts of C 2 H 6 , C 2 H 4 and CO 2 (denoted as MAF-49·C 2 H 6 , MAF-49·C 2 H 4 and MAF-49·CO 2 , respectively, see Supplementary Table 2 and Supplementary Data 3 , 4 , 5 ). Compared with the unit-cell volume of guest-free MAF-49, those of MAF-49·C 2 H 6 and MAF-49·C 2 H 4 showed minor shrinkage (<0.2%), while that of MAF-49·CO 2 showed relatively large expansion (1.4%). Further, the N8···C3 separation order of MAF-49, MAF-49·C 2 H 6 , MAF-49·C 2 H 4 and MAF-49·CO 2 is consistent with that predicted by computational simulations ( Supplementary Fig. 10 ). In all host–guest crystal structures, the residue electron density peaks can be unambiguously found inside the narrow host channel neck ( Fig. 3g–i ). Furthermore, in the final crystal structures, all guest molecules locate very similar or identical with those predicted by computational simulations ( Supplementary Fig. 10 ). Mixed gas separation To investigate the practical separation performance of MAF-49, breakthrough experiments were carried out at 313 K and 1 bar. 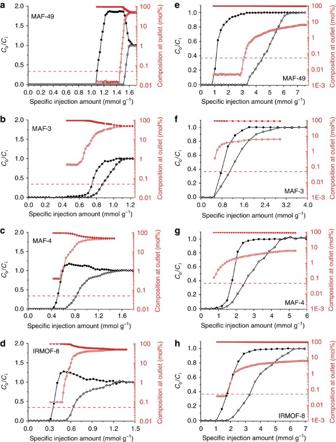Figure 5: C2H4/C2H6separation performances. C2H4/C2H6(1:1) mixture breakthrough curves of (a) MAF-49, (b) MAF-3, (c) MAF-4 and (d) IRMOF-8, and C2H4/C2H6(15:1) mixture breakthrough curves of (e) MAF-49, (f) MAF-3, (g) MAF-4 and (h) IRMOF-8 measured at 313 K and 1 bar. Solid symbols: C2H4, Open symbols: C2H6. Lines are drawn to guide eyes.CiandCoare the concentrations of each gas at the inlet and outlet, respectively. Horizontal red dashed lines highlight C2H6composition at outlet of 0.05%, that is, C2H4purity of 99.95%. To evaluate and compare the performances of the materials unambiguously, identical column and flow rate were used, and the parameters of each column were optimized (all columns have similar voidage, Supplementary Table 5 ). Besides, we used the specific injection amount (mmol g –1 ) of the mixed gas as the abscissa, meaning that the breakthrough time (s) was not only divided by the adsorbent weight (g) but also multiplied by the flow rate of the injected mixed gas (mmol s –1 ) [40] . To compare the gas adsorption and separation properties of MAF-49 with other protopytical MOFs, breakthrough experiments using an equimolar C 2 H 6 /C 2 H 4 /CO 2 /CH 4 mixture injection were carried out ( Fig. 4 and Supplementary Figs 11 and 12 ). For MAF-49, a clean and sharp separation of all four gases was observed, while other MOFs showed much poor separation performances and complicated effluent sequences dependent on their pore surface structures. With transition-metal OMSs, [Cu 3 (btc) 2 ] (HKUST-1, H 3 btc=benzene-1,3,5-tricarboxylic acid) and [Co 2 (dobdc)] (MOF-74-Co/CPO-27-Co, H 4 dobdc=2,5-dihydroxyl-1,4-benzenedicarboxylic acid) showed binding strength orders C 2 H 4 >C 2 H 6 >CO 2 . Because the main-group-metal OMS tends to form strong interaction with the oxygen atom of CO 2 , [Mg 2 (dobdc)] (MOF-74-Mg/CPO-27-Mg) showed a binding strength order CO 2 >C 2 H 4 >C 2 H 6 . Without pore surface active site, [Zr 6 O 4 (OH) 4 (bdc) 12 ] (UiO-66, H 2 bdc=1,4-benzenediarboxylic acid) and [Zn(mim) 2 ] (MAF-4 or ZIF-8, Hmim=2-methylimidazole) can barely distinguish the three heavier gases. Nevertheless, the low-polarity adsorbent MAF-4 exhibits slightly better performance compared with UiO-66, and exhibits a separation order similar with that of MAF-49. As expected from the analyses of adsorption isotherms, MAF-49 can also clearly separate two-component C 2 H 4 /C 2 H 6 , C 2 H 6 /CO 2 and C 2 H 6 /CH 4 mixtures ( Supplementary Fig. 13 ). It should be noted that C 2 H 6 could not be detected before its breakthrough points, meaning that C 2 H 6 is efficiently extracted and high-purity C 2 H 4 /CO 2 /CH 4 can be obtained directly. Figure 4: Four-component gas mixture separation. Breakthrough curves of CH 4 /CO 2 /C 2 H 4 /C 2 H 6 mixture (1:1:1:1 (vol)) for ( a ) CPO-27-Mg, ( b ) CPO-27-Co, ( c ) MAF-4, ( d ) UiO-66, ( e ) HKUST-1 and ( f ) MAF-49 measured at 313 K and 1 bar. Lines are drawn to guide eyes. C i and C o are the concentrations of each gas at the inlet and outlet, respectively. Full size image Considering that selective adsorption of C 2 H 6 over C 2 H 4 could be beneficial for purification of C 2 H 4 under fixed-bed adsorption/breakthrough processes, and some hydrophobic MOFs [29] , [30] , [31] , [32] , [33] , [34] , [35] , [36] , such as [Zn(bim) 2 ] (MAF-3 or ZIF-7, Hbim=benzimidazole), MAF-4 and [Zn 4 O(ndc) 3 ] (IRMOF-8, H 2 ndc=naphthalene-2,6-dicarboxylic acid), were recently reported to exhibit such a property, we compared the C 2 H 4 /C 2 H 6 adsorption and separation properties of these MOFs with MAF-49 in detail. Single-component C 2 H 6 adsorption isotherms were measured for MAF-3, MAF-4 and IRMOF-8, which show adsorption enthalpies of 25 kJ mol −1 , 18 kJ mol −1 and 30 kJ mol −1 , respectively ( Fig. 2c and Supplementary Fig. 14 ), at zero loading, being much lower than that of MAF-49. Although the C 2 H 6 uptake at 1 bar for MAF-49 (38 cm 3 g −1 ) is lower than that of the more porous adsorbents IRMOF-8 (91 cm 3 g −1 ), MAF-4 (48 cm 3 g −1 ) and MAF-3 (41 cm 3 g −1 ), its C 2 H 6 uptake at 0.06 bar (36 cm 3 g −1 ) is ca . 4 times that of IRMOF-8 (9 cm 3 g −1 ), 19 times that of MAF-4 (1.9 cm 3 g −1 ) and 45 times that of MAF-3 (0.8 cm 3 g −1 ) ( Fig. 2d ). Considering that a purity of 100% is impossible and the C 2 H 6 concentration before its breakthrough point is lower than the detection limit of the conventionally used thermal conductivity detector, the gas stream at the column outlet was analysed with a mass spectrometer (MS). For a 1:1 C 2 H 4 /C 2 H 6 mixture injection ( Fig. 5a and Supplementary Fig. 15a ), the breakthrough points of C 2 H 4 and C 2 H 6 for MAF-49 were observed by thermal conductivity detector at 1.09 and 1.44 mmol g −1 , respectively, during which the C 2 H 6 concentration was determined as 0.014–0.016% by MS, corresponding to a C 2 H 4 purity of 99.986–99.984% ( Fig. 5a and Supplementary Figs 15a and 16 ). Under identical conditions, the highest C 2 H 4 purities achieved by MAF-3, MAF-4 and IRMOF-8 are only 99.5%, 99.6% and 99.9% (C 2 H 6 concentrations of 0.5%, 0.4% and 0.1%), respectively, reflecting their much lower C 2 H 6 /C 2 H 4 selectivity compared with MAF-49 ( Fig. 5b–d , Supplementary Table 6 and Supplementary Figs 15–19 ). Nevertheless, such C 2 H 4 purities are obviously higher than those reported for C 2 H 4 selective adsorbent materials (99%+) [13] , [17] , [23] , [24] , which exemplify the feasibility of using C 2 H 6 selective adsorbents for purifying C 2 H 4 , because the desired gas can be continuously purified by passing through the column and directly obtained from the first effluents. Indeed, desorbing the MAF-49 column saturated by 1:1 C 2 H 4 /C 2 H 6 mixture can give C 2 H 6 with 99%+ purity with a peak value of only 99.7% ( Supplementary Fig. 20 ). A realistic comparison for the C 2 H 4 purification performance of different adsorbents, of relevance to industrial operations, can be obtained by comparing the breakthrough amount of C 2 H 4 (denoted as productivity) with the desired purity in a single breakthrough operation (for the calculation method see Supplementary Methods ). For the MAF-49 column, 0.28 mmol g −1 or 0.44 mol l −1 of C 2 H 4 with 99.95%+ purity can be recovered from a 1:1 C 2 H 4 /C 2 H 6 mixture injection. For the MAF-3, MAF-4 and IRMOF-8 columns, their productivities are zero because the C 2 H 4 effluents are not pure enough. Even for a C 2 H 4 purity of 99%+, the productivity of the MAF-49 column (0.32 mmol g −1 or 0.47 mol l −1 ) is still much higher than the others (the largest value is 0.11 mmol g −1 or 0.10 mol l −1 ) ( Supplementary Table 6 ). Figure 5: C 2 H 4 /C 2 H 6 separation performances. C 2 H 4 /C 2 H 6 (1:1) mixture breakthrough curves of ( a ) MAF-49, ( b ) MAF-3, ( c ) MAF-4 and ( d ) IRMOF-8, and C 2 H 4 /C 2 H 6 (15:1) mixture breakthrough curves of ( e ) MAF-49, ( f ) MAF-3, ( g ) MAF-4 and ( h ) IRMOF-8 measured at 313 K and 1 bar. Solid symbols: C 2 H 4 , Open symbols: C 2 H 6 . Lines are drawn to guide eyes. C i and C o are the concentrations of each gas at the inlet and outlet, respectively. Horizontal red dashed lines highlight C 2 H 6 composition at outlet of 0.05%, that is, C 2 H 4 purity of 99.95%. Full size image Since the C 2 H 6 concentration in C 2 H 4 /C 2 H 6 mixtures produced by hydrocarbon cracking is just ca . 5–9% (refs 41 , 42 , 43 ), breakthrough experiments using a 15:1 C 2 H 4 /C 2 H 6 mixture injection were carried out. The lowest C 2 H 6 impurity or highest C 2 H 4 purities achieved by the MAF-49, MAF-3, MAF-4 and IRMOF-8 columns are decreased to 0.005%, 0.4%, 0.1% and 0.04% or improved to 99.995%, 99.6%, 99.9% and 99.96%, respectively ( Fig. 5e–h and Supplementary Figs 21–24 ). Obviously, using C 2 H 6 selective adsorbents, the C 2 H 4 purity can be increased by lengthening the adsorbent bed (increasing adsorbent amount), which is simpler and more convenient than the C 2 H 4 selective adsorbents [13] , [17] , [25] . For the 15:1 C 2 H 4 /C 2 H 6 mixture injection and the C 2 H 4 output purity of 99.95%+, the MAF-49 column gave a C 2 H 4 productivity of 1.68 mmol g −1 or 2.48 mol l −1 , which is about 30 or 50 times that of IRMOF-8 (0.06 mmol g −1 or 0.05 mol l −1 ), in the gravimetric or volumetric point-of-view, respectively ( Supplementary Table 7 ). Note that for C 2 H 4 purification, the adsorbent volume is more practical than its weight because the fixed-bed equipment does not need to move during operation. For lower C 2 H 4 purities such as 99.5%+ and 99%+, the C 2 H 4 productivities of MAF-49 and IRMOF-8 were also increased ( Supplementary Tables 6 and 7 ), because the adsorber needs more time to reach adsorption saturation for the mixture gas containing low-concentration C 2 H 6 . Nevertheless, the C 2 H 4 productivity of MAF-49 improved more significantly than for IRMOF-8 at all purity standards ( Supplementary Tables 6 and 7 ), because the former material exhibits much higher C 2 H 6 uptakes at the low pressure region ( Fig. 2c ). In contrast, the MAF-3 and MAF-4 columns only showed slightly increased C 2 H 4 purities (did not reach 99.95%+) at a C 2 H 4 /C 2 H 6 feeding ratio of 15:1 ( Fig. 2c ), because lengthening the adsorber is not so effective to improve the effluent purity by using adsorbents with weak impurity affinity. For C 2 H 4 purities of 99.5%+ and 99%+, the C 2 H 4 productivities of the MAF-3 and MAF-4 columns obtained by using a 15:1 C 2 H 4 /C 2 H 6 input were unexpectedly lower than for the 1:1 C 2 H 4 /C 2 H 6 mixture ( Supplementary Tables 6 and 7 ), which can be attributed to the extremely low C 2 H 6 adsorption ability of the adsorbents at the low pressure region. Also, the partial pressures of C 2 H 4 and C 2 H 6 in the 15:1 C 2 H 4 /C 2 H 6 mixture are not beneficial for utilizing the differential gate-opening effect of MAF-3 (ref. 44 ). In summary, we reported a unique adsorbent material showing selective adsorption of C 2 H 6 over more polar analogous molecules such as C 2 H 4 and CO 2 , which can be useful for extraction of C 2 H 6 from natural gases and particularly valuable for direct production of high-purity C 2 H 4 from C 2 H 4 /C 2 H 6 mixtures. The key to this C 2 H 6 selectivity is a combination of multiple hydrogen-bonding acceptors and dipole repulsion groups locating at appropriate positions on the pore surface of a very narrow channel, which not only allows multiple attractive interactions for C 2 H 6 but also enforces C 2 H 4 to adopt a position that can only form fewer and weaker attractive interactions. In short, this work provides not only a new MOF with exceptionally high C 2 H 4 separation/purification performances, but also a new molecular design strategy for developing next-generation adsorbents. Materials and general methods Reagents and solvents were commercially available and were used without further purification, H 2 batz (ref. 45 ), MAF-3 (ref. 30 ), MAF-4 (ref. 46 ), IRMOF-8 (ref. 47 ), HKUST-1 (ref. 48 ), CPO-27-Mg (ref. 49 ), CPO-27-Co (ref. 49 ) and UiO-66 (ref. 50 ) were synthesized according to the literature methods. Elemental analyses (C, H, N) were performed with a Vario EL elemental analyzer. Thermogravimetry analysis was performed under N 2 with temperature increased with 5 °C min –1 using a TA-Q50 system. Powder XRD patterns were collected on a Bruker D8 Advance diffractometer (Cu Kα) at room temperature. Synthesis of [Zn(batz)]·0.5H 2 O (MAF-49·H 2 O) A mixture of Zn(OH) 2 (0.100 g, 1.0 mmol), H 2 batz (0.180 g, 1.0 mmol), aqueous ammonia (25%, 4 ml) and water (4 ml) was stirred for 15 min in air, then transferred and sealed in a 15 ml Teflon reactor, which was heated in an oven at 160 °C for 72 h. The oven was cooled to room temperature at a rate of 5 °C h −1 . The resulting colourless block crystals were filtered, washed and dried in air (yield ca . 86%). Anal. Calcd (%) for C 5 H 7 N 8 O 0.5 Zn: C, 23.77; H, 2.79; N, 44.36. Found: C, 23.97; H, 2.82; N, 44.13. Guest-free MAF-49 was obtained by heating the as-synthesized sample under high vacuum at 150 °C for 12 h. Single-crystal X-ray crystallography Diffraction intensities were collected on a Pilatus XtaLAB P300DS diffractometer with graphite-monochromated Mo Kα radiation. Absorption corrections were applied by using the multi-scan programme REQAB. The structures were solved by the direct method and refined with the full-matrix least-squares technique using the SHELXTL programme package. It should be noted that, because the molecular centres of the very short C 2 H 6 and C 2 H 4 molecules do not locate at the centre of the two-fold symmetric host channel neck as predicted by computational simulations, their molecular geometries have to be restricted during refinement of the crystal structures. Also, the positions of their hydrogen atoms were added according to the computational simulation result. Because of disorder and low occupancies of the gas molecules, anisotropic thermal parameters were only applied to all non-hydrogen atoms of the host framework. Crystal data for the compounds were summarized in Supplementary Table 2 . Electron density maps were generated using the output from standard SHELXL refinements in a number of ways using WinGX and VESTA 3.0.8. Gas sorption measurement The sorption isotherms were measured with an automatic volumetric adsorption apparatus (BELSORP-max). The as-synthesized sample (about 200−300 mg) was placed in the sample tube and dried for 12 h at 320 °C to remove the remnant solvent molecules prior to measurement. CO 2 (99.999%), C 2 H 4 (99.95%), CH 4 (99.999%) and C 2 H 6 (99.99%) were used for all adsorption isotherm and breakthrough experiments ( Supplementary Fig. 25 ). The temperatures were controlled by a water bath (298, 307 and 316 K). Accession codes: The X-ray crystallographic coordinates for structures reported in this Article have been deposited at the Cambridge Crystallographic Data Centre (CCDC), under deposition number CCDC 1421354-1421358. These data can be obtained free of charge from the Cambridge Crystallographic Data Centre via www.ccdc.cam.ac.uk/data_request/cif . How to cite this article: Liao, P.-Q. et al . Efficient purification of ethene by an ethane-trapping metal-organic framework. Nat. Commun. 6:8697 doi: 10.1038/ncomms9697 (2015).